A recently evolved class of alternative 3′-terminal exons involved in cell cycle regulation by topoisomerase inhibitors Alternative 3′-terminal exons, which use intronic polyadenylation sites, are generally less conserved and expressed at lower levels than the last exon of genes. Here we discover a class of human genes, in which the last exon appeared recently during evolution, and the major gene product uses an alternative 3′-terminal exon corresponding to the ancestral last exon of the gene. This novel class of alternative 3′-terminal exons are downregulated on a large scale by doxorubicin, a cytostatic drug targeting topoisomerase II, and play a role in cell cycle regulation, including centromere–kinetochore assembly. The RNA-binding protein HuR/ELAVL1 is a major regulator of this specific set of alternative 3′-terminal exons. HuR binding to the alternative 3′-terminal exon in the pre-messenger RNA promotes its splicing, and is reduced by topoisomerase inhibitors. These findings provide new insights into the evolution, function and molecular regulation of alternative 3′-terminal exons. Most human genes generate alternative transcripts through the use of alternative splice sites (90% genes), promoters (60%) and cleavage-and-polyadenylation (polyA) sites (60%). Large numbers of alternatively spliced exons are coordinately regulated during various processes, including notably cell differentiation and cancer [1] , [2] , but studies mainy focused on cassette exons. Likewise, alternative polyA sites are widely regulated during several processes, most notably cell proliferation, where shorter forms are preferentially expressed [3] , [4] , [5] , [6] , [7] , but studies mainly focused on tandem polyA sites, which are located in the same exon. Thus, little is known about the regulation of alternative 3′ terminal exons, also called alternative last exons (ALEs), which are found in >3,000 human genes and correspond to the alternative use of intronic polyA sites in a splicing-dependent manner [7] , [8] , [9] . In contrast with tandem polyA sites, which are located within 3′UTRs, intronic polyA sites affect coding regions and give rise to protein isoforms. In some genes, ALE isoforms have specialized functions (for example, IgM heavy chain and CT-CGRP genes) [8] . However, in general the 3′-most exon of a gene (referred to as the last ALE in this study) is viewed as producing the full-length isoform, while internal ALEs lead to less abundant and truncated isoforms, sometimes with dominant-negative properties [10] , [11] , [12] . Consistently, intronic polyA sites are much less conserved between human and murine cDNAs when compared with 3′-most polyA sites [9] , [13] . Moreover, many cryptic polyA sites lie in introns and are silenced by a mechanism called telescripting [11] , [12] . ALEs are widely regulated in a tissue-specific manner [14] , but little is known about their dynamic regulation. Interestingly, internal ALEs are preferentially upregulated during neuron activation [15] ; a similar regulation was found during cell proliferation in one study [6] , but not in another [5] . Thus, little is known about ALE regulation on a large scale. One biological setting where alternative transcripts are emerging as important new players is the response of cells to DNA-damaging agents [16] . These responses involve a partial repression of gene expression, accompanied by the selective upregulation of genes involved in DNA repair, cell cycle arrest and eventually cell death, which is coordinated in a large part by the p53 transcription factor. Likewise, UV irradiation partially inhibits cleavage/polyadenylation [17] , but p53 transcripts escape such repression [18] . Several genes involved in the DNA damage response, such as MDM2 that encodes the main repressor of p53, are regulated at the splicing level in response to genotoxic agents [16] . Recently, UV irradiation and the topoisomerase (TOP) I inhibitor, camptothecin (CPT), were shown to increase the inclusion of many cassette exons through an inhibition of transcription elongation, which gives more time for the cotranscriptional recognition and inclusion of alternative exons [19] , [20] , [21] . CPT also induces skipping of a set of exons, in part by disrupting the interaction between the EWS and YB-1 proteins [22] . However, CPT, the only genotoxic agent that was studied for exonic regulations on a genome-wide scale, can inhibit transcription elongation independently of DNA damage [23] . Moreover, other types of alternative exons such as ALEs were not examined in these studies. Interestingly, a recent study in yeast showed that DNA damage can affect polyA site use in many genes [24] . Thus, additional large-scale analyses of the effects of genotoxic agents on alternative transcripts are needed. Doxorubicin (DOXO), the main drug used in breast cancer chemotherapy, is a TOP-II inhibitor that induces double-strand DNA breaks but does not otherwise inhibit transcription elongation [23] . A few cases of splicing regulation by TOP-II inhibitors were previously reported [22] , [25] , [26] , [27] . Here using a genome-wide approach, we show that ALEs are the main type of exons regulated by acute DOXO treatment in a breast cancer cell line. Given the high prevalence and highly specific pattern of ALE regulation by DOXO, we then determine the functional impact and molecular mechanism of this regulation. Our findings identify a class of evolutionarily recent ALEs that are regulated on a large scale by DOXO, identify the RNA-binding protein HuR/ELAVL1 as a regulator of ALE maturation in response to TOP inhibitors, and implicate ALEs in cell cycle regulation and chemotherapy. ALEs are a major type of exons regulated by TOP inhibitors To identify alternative exons regulated by DOXO in the MCF-7 breast cancer cell line, we used pan-genomic exon-arrays. We also compared the effects of DOXO and CPT, which we analysed in the same cell line using the same technology [22] . Drug treatments were done for only 6 h to identify regulations that are not a consequence of toxicity. Exon-array data were analysed using the splicing index method followed by manual curation. We identified 248 exons regulated by DOXO by >1.8-fold (Student’s paired t -test, P <0.05; Supplementary Data 1 ). By RT-PCR analysis we validated 37 exonic regulations (validation rate of 62%; Fig. 1e and Supplementary Fig. 1 ). Meanwhile, 333 genes were regulated at the global level by >1.8-fold (Student’s paired t -test, P <0.05; Supplementary Data 2 ). Most of the exonic regulations we identified did not occur in globally regulated genes ( Fig. 1a and Supplementary Fig. 1e ). 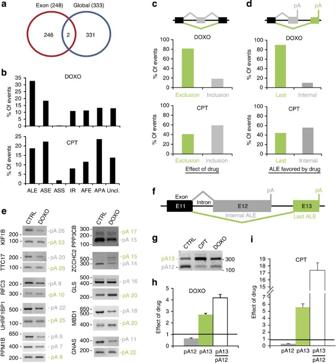Figure 1: Repression of internal ALEs is a major type of exon regulation by DOXO. (a) Venn diagram of genes regulated by DOXO at the exon or global levels. (b) Classification of alternative exons regulated by DOXO or CPT. ALE, alternative last exons; ASE, cassette exons; ASS, alternative splice sites; IR, intron retention; AFE, alternative first exons (alternative promoters); APA, tandem polyA sites; Uncl., unclassified. (c) Effects of DOXO and CPT on cassette exons (exclusion or inclusion). (d) Effects of DOXO and CPT on the internal ALE/last ALE ratio. In (candd), a test of proportions shows that DOXO more often induces exon exclusion (or last-ALE induction) than CPT (P<4.10−4andP<6.10−7, respectively). (e) RT–PCR validation of ALE regulation by DOXO. Isoforms are designated by ‘pA’ and exon number. The location of size markers (in bp) is indicated. Representative data of three independent experiments are shown. (f) Schematics of theCENPNgene. Exons and introns are represented by rectangles and lines, respectively. pA, polyA site. (g–i) Regulation of ALEs by DOXO and CPT in theCENPNgene. Analysis by RT-PCR (g) and RT-qPCR (h,i). Data represent the mean±s.e.m. of 16 (h) or 5 (i) independent experiments. All drug treatments were done for 6 h. CTRL, vehicle-treated cells. However, both sets were enriched in genes involved in cell cycle ( Table 1 ), suggesting that exon regulations, like global gene regulations, may play a role in cellular responses to DOXO (see below). Figure 1: Repression of internal ALEs is a major type of exon regulation by DOXO. ( a ) Venn diagram of genes regulated by DOXO at the exon or global levels. ( b ) Classification of alternative exons regulated by DOXO or CPT. ALE, alternative last exons; ASE, cassette exons; ASS, alternative splice sites; IR, intron retention; AFE, alternative first exons (alternative promoters); APA, tandem polyA sites; Uncl., unclassified. ( c ) Effects of DOXO and CPT on cassette exons (exclusion or inclusion). ( d ) Effects of DOXO and CPT on the internal ALE/last ALE ratio. In ( c and d ), a test of proportions shows that DOXO more often induces exon exclusion (or last-ALE induction) than CPT ( P <4.10 −4 and P <6.10 −7 , respectively). ( e ) RT–PCR validation of ALE regulation by DOXO. Isoforms are designated by ‘pA’ and exon number. The location of size markers (in bp) is indicated. Representative data of three independent experiments are shown. ( f ) Schematics of the CENPN gene. Exons and introns are represented by rectangles and lines, respectively. pA, polyA site. ( g – i ) Regulation of ALEs by DOXO and CPT in the CENPN gene. Analysis by RT-PCR ( g ) and RT-qPCR ( h , i ). Data represent the mean±s.e.m. of 16 ( h ) or 5 ( i ) independent experiments. All drug treatments were done for 6 h. CTRL, vehicle-treated cells. Full size image Table 1 DOXO-regulated exons are enriched in cell cycle genes. Full size table We then compared the large-scale patterns of exon regulation by DOXO and CPT, using the identified top-lists of regulated exons for each drug ( Supplementary Data 1 and 3 ). Interestingly, ALEs were the most prominent category of exons regulated by DOXO, and a major category of exons regulated by CPT (almost as frequent as cassette exons; Fig. 1b ). Regulations of cassette exons may be over-estimated because there are many more cassette exons than ALEs in transcript databases and exon-arrays. In addition, the splicing index method was originally designed for cassette exons and may not be optimal for mutually exclusive exons such as ALEs. Using an algorithm specifically comparing the regulation of internal ALEs to their following exon, we identified additional ALEs regulated by DOXO ( Supplementary Data 4 ). In total, we identified 100 genes regulated by DOXO at the level of ALEs (both ‘skipped ALEs’ and ‘composite ALEs’; see methods). Extensive RT-PCR validations are shown in Fig. 1e and Supplementary Fig. 1c,d . Thus, ALEs are a major category of alternative exons regulated by both TOP-I and TOP-II inhibitors. DOXO preferentially represses internal ALEs As expected from previous studies and from its ability to inhibit transcription elongation [20] , [21] , [22] , CPT favored inclusion more often than exclusion of cassette exons ( Fig. 1c ). Likewise, CPT favored the expression of the internal ALE slightly more often than the last ALE (56 versus 44% cases; Fig. 1d ). On the other hand, strikingly, DOXO favored the exclusion of cassette exons in 82% cases ( Fig. 1c ), which is significantly more often than CPT ( P <4.10 −4 , test of proportions). Likewise, DOXO favored the expression of the last ALE in 90% of cases ( Fig. 1d ), which is significantly more often than CPT ( P <6.10 −7 , test of proportions). The CPT-specific effects will be discussed below (see Discussion). Altogether, internal ALE repression appears to be the main exonic effect of DOXO, and is also a highly prevalent effect of CPT ( Fig. 1b,d ). We validated 23 such regulations by RT-PCR for DOXO ( Fig. 1e and Supplementary Fig. 1c,d ). We also validated by RT-PCR several cases of internal ALE repression that were predicted to be induced by both drugs ( Supplementary Fig. 1d and Supplementary Data 5 ). For example, the CENPN gene generates CENPN-pA12 transcripts ending in exon 12 (E12), and CENPN-pA13 transcripts skipping E12 and ending in E13 ( Fig. 1f ). Competitive RT–PCR analysis indicates that CENPN-pA12 is the major isoform in untreated cells, whereas CENPN-pA13 is the major isoform after DOXO or CPT treatment for 6 h ( Fig. 1g ). Quantitative RT-PCR analysis indicates that DOXO and CPT increase the CENPN-pA13/CENPN-pA12 isoform ratio by 4.3- and 17.4-fold, respectively, by decreasing CENPN-pA12 while increasing CENPN-pA13 levels ( Fig. 1h,i ). Meanwhile, total CENPN mRNA level was not affected by DOXO and only moderately decreased by CPT ( Supplementary Fig. 2a ). The regulation of ALE isoforms by DOXO and CPT was verified at later time points (with stronger effects at 24 h) and in another breast cancer cell line ( Supplementary Fig. 2b–e ). DOXO represses internal ALEs corresponding to major isoforms Internal ALEs are often considered to correspond to low-abundance truncated variants, and last ALEs to major full-length isoforms [10] , [11] , [12] . However, we found that DOXO-repressed internal ALEs correspond to highly expressed isoforms. Indeed, RT–PCR analysis of untreated cells detected higher levels of the DOXO-repressed internal ALE isoform than the last-ALE isoform in 9 out of 11 tested genes ( Figs 1g and 2a ). Consistently, in transcript databases, the fraction of transcripts ending at the internal ALE is higher for genes where DOXO represses the internal ALE, when compared with other genes with ALEs in the genome ( Fig. 2b ). Moreover, exon-array data in untreated cells indicated that gene-normalized expression was lower in the case of DOXO-induced last ALEs, when compared with other last ALEs in the genome ( Fig. 2c ). Thus, DOXO-repressed internal ALEs correspond to highly expressed, often major isoforms ( Fig. 2a ), whereas for most human genes the last ALE corresponds to the major isoform. 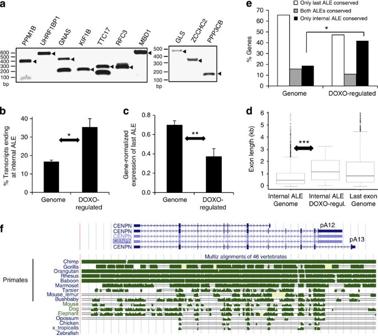Figure 2: DOXO represses internal ALEs corresponding to major isoforms. (a) Competitive RT–PCR amplification of internal and last-ALE isoforms in untreated cells. Arrowheads indicate internal ALE isoforms. Last-ALE isoforms are often not detected, although they can be amplified separately as shown inFig. 1e. The location of size markers (in bp) is indicated. Representative data of three independent experiments are shown. (b) Percent of transcripts from Genbank that end at the internal ALE rather than the last ALE, in genes whose ALEs are regulated by DOXO (internal ALE repression) or not. Shown are medians±s.e.m. of 50 and 1,545 genes, respectively (see Methods). (c) Gene-normalized expression of last ALEs that are regulated by DOXO (upregulation relative to internal ALE) or not. Exon-array data from untreated cells. Shown are medians±s.e.m. of 38 and 304 genes, respectively (see methods). (d) Boxplot of exon length, comparing DOXO-repressed internal ALEs (n=48) with internal and last ALEs in the genome (n=2,216). Shown are the median, the first and third quartiles, 1.5 times the interquartile range (whiskers) and outliers. (e) Conservation of human ALEs in non-mammalian vertebrates. Comparison of DOXO-regulated ALEs and randomly selected control ALEs (n=55 and 32, respectively; see Methods). (f) Multi-alignment of theCENPNgene sequence in various Vertebrates (screenshot from the UCSC genome browser; green areas are conserved regions). *P<5.10−2; **P<5.10−4and ***P<2.10−5. Wilcoxon rank sum test (b–d) or test of proportions (e). Figure 2: DOXO represses internal ALEs corresponding to major isoforms. ( a ) Competitive RT–PCR amplification of internal and last-ALE isoforms in untreated cells. Arrowheads indicate internal ALE isoforms. Last-ALE isoforms are often not detected, although they can be amplified separately as shown in Fig. 1e . The location of size markers (in bp) is indicated. Representative data of three independent experiments are shown. ( b ) Percent of transcripts from Genbank that end at the internal ALE rather than the last ALE, in genes whose ALEs are regulated by DOXO (internal ALE repression) or not. Shown are medians±s.e.m. of 50 and 1,545 genes, respectively (see Methods). ( c ) Gene-normalized expression of last ALEs that are regulated by DOXO (upregulation relative to internal ALE) or not. Exon-array data from untreated cells. Shown are medians±s.e.m. of 38 and 304 genes, respectively (see methods). ( d ) Boxplot of exon length, comparing DOXO-repressed internal ALEs ( n =48) with internal and last ALEs in the genome ( n =2,216). Shown are the median, the first and third quartiles, 1.5 times the interquartile range (whiskers) and outliers. ( e ) Conservation of human ALEs in non-mammalian vertebrates. Comparison of DOXO-regulated ALEs and randomly selected control ALEs ( n =55 and 32, respectively; see Methods). ( f ) Multi-alignment of the CENPN gene sequence in various Vertebrates (screenshot from the UCSC genome browser; green areas are conserved regions). * P <5.10 −2 ; ** P <5.10 −4 and *** P <2.10 −5 . Wilcoxon rank sum test ( b – d ) or test of proportions ( e ). Full size image DOXO-repressed internal ALEs resemble more last exons of genes than average internal ALEs, not only according to expression level but also to exon length, as they were on average longer than other internal ALEs in the human genome, like last ALEs ( Fig. 2d ). Consistently, DOXO-repressed internal ALEs often correspond to ancestrally last exons of genes. Indeed, while for randomly selected human genes, the internal ALE rarely corresponds to the last exon of the gene in non-mammalian vertebrates ( Fig. 2e , ‘genome’), DOXO-repressed internal ALEs correspond to the ancestral last exon of the gene in ~50% cases ( Fig. 2e , ‘DOXO-regulated’). The novel last ALE appeared either in mammals (in most cases) or in primates (example in Fig. 2f ). Thus, DOXO-repressed internal ALEs are strongly enriched in a particular class of internal ALEs that are highly expressed and correspond to ancestrally last exons and therefore full-length isoforms. Further supporting this notion, in several cases (including UHRF1BP1 ; Supplementary Fig. 1f ) the last-ALE isoform bears a premature stop codon, which is known to induce nonsense-mediated mRNA decay (NMD) instead of productive translation. As NMD isoforms are expected to be expressed at low levels even after splicing induction, we re-analysed our exon-array data with relaxed stringency on exon expression, and found 16 additional genes with DOXO-induced last ALEs of the NMD type. Altogether, our data indicate that DOXO typically represses internal ALEs that encode abundant (often major) and ancestrally full-length isoforms, suggesting that this regulation may have a functional impact. DOXO-regulated ALEs play a role in cell cycle regulation As already mentioned, DOXO-regulated exons were enriched in genes involved in DNA damage response (including DNA repair) and cell cycle, more specifically M phase-associated processes (for example, chromosome and centromere–kinetochore–spindle network; Table 1 ). Similar functions were enriched when focusing on DOXO-regulated ALEs ( Table 1 ). Enrichment in mitosis-related genes is also found in globally regulated genes ( Table 1 ) and is highly relevant because the inhibition of cell cycle progression (an important aspect of the DNA damage response) in response to DOXO mainly occurs at the level of G2/M (ref. 28 ). To test the role of DOXO-regulated ALEs in cell cycle regulation, we focused on the CENPN gene that is involved in centromere–kinetochore assembly and mitosis [29] . Assembly of the CCAN complex (Constitutive Centromere Associated Network) is directed by a centromere-specific histone variant called CENPA that recruits CENPN through interaction with CENPN N-terminal region ( Fig. 3a and Supplementary Fig. 3a ). In turn, CENPN recruits several other CCAN components (including CENPH) through interaction of its C-terminal region with CENPL [30] . However, only the CENPN-pA12 isoform, corresponding to the internal ALE and the ancestral isoform, has been studied. Interestingly, half of the CENPL-interacting region that was mapped [30] is absent in the CENPN-pA13 isoform. To test whether the CENPN-pA13 isoform is unable to promote CCAN assembly, we developed siRNAs targeting either both CENPN isoforms or each isoform selectively ( Fig. 3b and Supplementary Fig. 3b ). 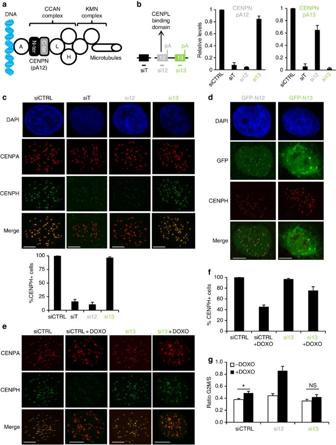Figure 3: DOXO-regulated ALEs play a role in centromere–kinetochore assembly and cell cycle. (a) Schematics of the centromere–kinetochore network. (b) RT–qPCR validation of siRNAs targeting either both CENPN isoforms or each isoform selectively (48-hour transfection). Data represent the mean±s.e.m. of four independent experiments. (c) Immunofluorescence of CENPA and CENPH following transfection of siRNAs targeting CENPN isoforms for 48 h. CENPH data are quantified on the bottom panel. Data represent the mean±s.e.m. of five independent experiments. (d) (Immuno-) fluorescence of GFP and CENPH following transfection of GFP-CENPN isoform constructs for 24 h. Representative data of four independent experiments are shown. (e,f) Immunofluorescence of CENPA and CENPH following transfection with siCTRL or si13 for 48 h, including 19 h with or without DOXO. Data are quantified in (f). Data represent the mean±s.e.m. of three independent experiments. (g) FACS analysis of cell cycle (G2M:S ratio) following transfection of siRNAs targeting CENPN isoforms for 48 h, including 19 h with or without DOXO. Data represent the mean±s.e.m. of seven independent experiments. *P<2.10−2(Student’s pairedt-test). NS, not significant. siCTRL, siRNA targeting luciferase; siT, siRNA targeting both CENPN isoforms. In (c–e), scale bars represent 5 μm. Figure 3: DOXO-regulated ALEs play a role in centromere–kinetochore assembly and cell cycle. ( a ) Schematics of the centromere–kinetochore network. ( b ) RT–qPCR validation of siRNAs targeting either both CENPN isoforms or each isoform selectively (48-hour transfection). Data represent the mean±s.e.m. of four independent experiments. ( c ) Immunofluorescence of CENPA and CENPH following transfection of siRNAs targeting CENPN isoforms for 48 h. CENPH data are quantified on the bottom panel. Data represent the mean±s.e.m. of five independent experiments. ( d ) (Immuno-) fluorescence of GFP and CENPH following transfection of GFP-CENPN isoform constructs for 24 h. Representative data of four independent experiments are shown. ( e , f ) Immunofluorescence of CENPA and CENPH following transfection with siCTRL or si13 for 48 h, including 19 h with or without DOXO. Data are quantified in ( f ). Data represent the mean±s.e.m. of three independent experiments. ( g ) FACS analysis of cell cycle (G2M:S ratio) following transfection of siRNAs targeting CENPN isoforms for 48 h, including 19 h with or without DOXO. Data represent the mean±s.e.m. of seven independent experiments. * P <2.10 −2 (Student’s paired t -test). NS, not significant. siCTRL, siRNA targeting luciferase; siT, siRNA targeting both CENPN isoforms. In ( c – e ), scale bars represent 5 μm. Full size image In untreated cells, CENPH colocalized with CENPA nuclear foci that mark centromeres, and this colocalization was strongly decreased by siRNAs targeting either both CENPN isoforms or CENPN-pA12 only ( Fig. 3c ), as expected from previous studies [29] , [30] , [31] . In contrast, CENPH colocalization with CENPA was not affected by several siRNAs targeting the CENPN-pA13 isoform selectively ( Fig. 3c and Supplementary Fig. 3c ). Moreover, CENPN isoforms exhibited different subcellular localization. Indeed, using GFP-CENPN constructs as in previous studies, the CENPN-pA12 isoform exhibited punctate staining strongly colocalizing with both CENPA and CENPH ( Fig. 3d and Supplementary Fig. 3d , ‘GFP-N12’), in addition to some diffuse staining as previously reported [30] , [32] . In contrast, the CENPN-pA13 isoform did not colocalize with CENPA or CENPH ( Fig. 3d and Supplementary Fig. 3d , ‘GFP-N13’), indicating a defect in centromere localization. This is consistent with the fact that CENPN association with centromeres is stabilized by its C-terminal domain ( Supplementary Fig. 3d , ‘GFP-N ΔC-ter’) [30] , [31] , [32] . Altogether, our data indicate that DOXO represses the expression of the CENPN-pA12 isoform that mediates centromere–kinetochore assembly, and increases the CENPN-pA13 isoform that is not competent for this activity. Consistently, DOXO disrupted (in 55% cells) the colocalization of CENPH with CENPA without affecting CENPA staining ( Fig. 3e,f ), similarly to CENPN-pA12 depletion. Interestingly, CENPN-pA13 depletion partially prevented the disruption of CENPH foci by DOXO ( Fig. 3e,f and Supplementary Fig. 3e ), suggesting a role of the CENPN-pA13 isoform in the presence of DOXO. These data reveal that DOXO disrupts CCAN assembly, at least in part through CENPN isoform switching. Furthermore, CENPN-pA12 depletion increased the accumulation of MCF-7 cells in G2/M in the presence of DOXO at a dose and time point where DOXO had only a modest effect by itself ( Fig. 3g ). This effect is consistent with the role of CENPN in mitosis through kinetochore assembly [29] . Conversely, the effect of DOXO on G2/M was partially prevented by CENPN-pA13 depletion, and this was more evident when using a dose of DOXO that has a stronger effect on G2/M accumulation ( Fig. 3g and Supplementary Fig. 3f ). Altogether, our data suggest that the CENPN-pA13 isoform does not promote CCAN assembly and G2/M progression, but may inhibit these processes in DOXO-treated cells ( Fig. 3c–g and Supplementary Fig. 3 ). Thus, DOXO-induced switch of CENPN isoforms may play a role in the regulation of centromere–kinetochore assembly and cell cycle by DOXO. TOP inhibitors repress internal ALEs at the pre-mRNA level Given the high prevalence and functional relevance of internal ALE repression by DOXO, we then investigated the underlying molecular mechanism, mainly focusing on the CENPN gene. As CPT also represses internal ALEs in a large set of genes ( Fig. 1d ), including CENPN ( Fig. 1g ), the effects of CPT were analysed in parallel to potentially identify mechanisms of internal ALE repression shared by TOP inhibitors. The differential regulation of ALE isoform expression could be due either to differential mRNA stability, because 3′UTRs can regulate cytoplasmic mRNA stability, or to the regulation of nuclear pre-mRNA maturation, as ALE selection depends on an interplay between alternative splicing and polyadenylation ( Fig. 4a ). Several data indicate that ALE isoform regulation by DOXO and CPT is mediated at least in part at the level of nuclear maturation. First, DOXO and CPT induced a switch of CENPN isoforms ( Fig. 1h,i ). Second and more importantly, the regulation was observed in the nucleus ( Fig. 4b ). Third, actinomycin D prevented the effect of DOXO on CENPN isoform ratio, indicating a requirement for on-going transcription, but did not affect the CENPN isoform ratio by itself, suggesting no differential isoform stability ( Fig. 4c ). Fourth, DOXO and CPT strongly increased the spliced to unspliced ratio of CENPN exon E13 in nuclear RNA fractions, without increasing the spliced to unspliced ratio of E12 ( Fig. 4d and Supplementary Fig. 2f ). Fifth, DOXO and CPT increased the use of the E13 polyA site relative to the E12 polyA site, as shown by quantifying in nuclear RNA fractions, the transcripts upstream and downstream of each polyA site [18] ( Supplementary Fig. 2g ). In addition to CENPN , we also verified for two other genes that the regulation of ALE isoforms by DOXO was observed in the nucleus ( Supplementary Fig. 2h ). However, we cannot exclude that for some other genes, or in addition to nuclear effects, DOXO might also affect cytoplasmic mRNA isoform stability, for example through miRNAs. 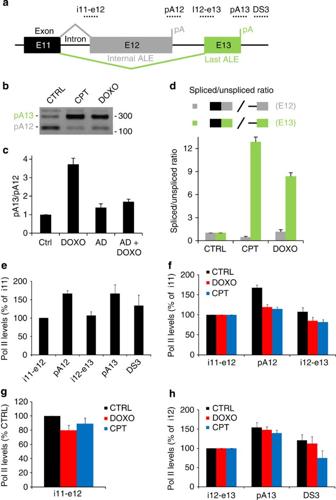Figure 4: TOP inhibitors affect ALE isoform expression at the level of pre-mRNA maturation. (a) Schematics of theCENPNgene. Exons and introns are represented by rectangles and lines, respectively. Amplicons used ine–hare shown. pA, polyA site. (b) RT–PCR analysis of CENPN isoform expression in nuclear RNA following drug treatment as indicated. The location of size markers (in bp) is indicated. Representative data of five independent experiments are shown. (c) RT–qPCR analysis of CENPN isoform ratio following treatment with DOXO and/or actinomycin D (‘AD’). Data represent the mean±s.e.m. of four independent experiments. (d) RT–qPCR analysis of nuclear RNA for the effects of drugs on the ratio of spliced to unspliced transcripts for each ALE of CENPN. Controls are set to 1. Data represent the mean±s.e.m. of four independent experiments. (e–h) Chromatin immunoprecipitation with an anti-Pol-II antibody followed by qPCR analysis of the indicated regions in theCENPNgene. Drug treatments are indicated. Note that DOXO and CPT had little effect on Pol-II levels at the level of i11-e12. Data represent the mean±s.e.m. of four independent experiments. All drug treatments were done for 6 h. Figure 4: TOP inhibitors affect ALE isoform expression at the level of pre-mRNA maturation. ( a ) Schematics of the CENPN gene. Exons and introns are represented by rectangles and lines, respectively. Amplicons used in e – h are shown. pA, polyA site. ( b ) RT–PCR analysis of CENPN isoform expression in nuclear RNA following drug treatment as indicated. The location of size markers (in bp) is indicated. Representative data of five independent experiments are shown. ( c ) RT–qPCR analysis of CENPN isoform ratio following treatment with DOXO and/or actinomycin D (‘AD’). Data represent the mean±s.e.m. of four independent experiments. ( d ) RT–qPCR analysis of nuclear RNA for the effects of drugs on the ratio of spliced to unspliced transcripts for each ALE of CENPN. Controls are set to 1. Data represent the mean±s.e.m. of four independent experiments. ( e – h ) Chromatin immunoprecipitation with an anti-Pol-II antibody followed by qPCR analysis of the indicated regions in the CENPN gene. Drug treatments are indicated. Note that DOXO and CPT had little effect on Pol-II levels at the level of i11-e12. Data represent the mean±s.e.m. of four independent experiments. All drug treatments were done for 6 h. Full size image As cleavage/polyadenylation is connected to transcription termination, and polyA sites induce RNA polymerase II (Pol-II) pausing [33] , we determined the impact of DOXO and CPT on Pol-II dynamics on the CENPN gene by chromatin immunoprecipitation. In untreated cells, we observed peaks of Pol-II levels around both E12 and E13 polyA sites compared with matched upstream regions ( Fig. 4e ), which is consistent with pauses of Pol-II occurring around each polyA site. DOXO and CPT strongly reduced the peak of Pol-II over the E12 polyA site compared with an upstream region ( Fig. 4f,g ), suggesting an inhibition of the recognition of this polyA site (or its ability to induce pausing) and reflecting the decrease of the CENPN-pA12 mRNA. In contrast, DOXO and CPT did not reduce the peak of Pol-II over the E13 polyA site ( Fig. 4h ). Altogether, these data suggest that DOXO and CPT inhibit the cotranscriptional recognition of the internal ALE in the CENPN gene. HuR/ELAVL1 mediates internal ALE repression by TOP inhibitors Looking for splicing- and polyadenylation-regulatory factors that may mediate ALE regulation in response to DOXO, we found ~20 factors whose expression anti-correlated with the inclusion rate of DOXO-stimulated last ALEs across a panel of human cell lines in a publicly available exon-array data set (ENCODE [34] ; Supplementary Data 6 ). Two of these factors were previously involved in DNA damage responses. The first one, BARD1, inhibits cleavage/polydenylation in response to UV irradiation [17] , [35] . As expected from the anti-correlation data, the CENPN-pA13/CENPN-pA12 ratio was increased following BARD1 depletion ( Supplementary Fig. 4a,b ). In addition, BARD1 depletion decreased the fold-effect of DOXO on the CENPN isoform ratio, but only by half ( Supplementary Fig. 4c ), and in fact, the isoform ratio measured in the presence of DOXO was not decreased by BARD1 depletion ( Supplementary Fig. 4d ). Thus, the effect of DOXO on CENPN ALEs appears to be only partially mediated by BARD1. The second factor, HuR/ELAVL1, is an RNA-binding protein that has long been involved in the regulation of cytoplasmic mRNA stability and translation in response to DNA damage (reviewed by Gorospe [36] ) and more recently in pre-mRNA splicing and polyA site use in the nucleus [37] , [38] , [39] , [40] , [41] , [42] . As expected from the anti-correlation data, the depletion of HuR using a specific siRNA in MCF-7 cells ( Fig. 5a ) led to an increase in the CENPN-pA13/CENPN-pA12 mRNA ratio ( Fig. 5b ). This result was confirmed using a second siRNA ( Supplementary Fig. 5a ). Importantly, HuR depletion impacted the CENPN isoform ratio in the nucleus ( Fig. 5c ) and increased the spliced to unspliced ratio of E13 but not E12 ( Fig. 5d ). Thus, HuR depletion affects CENPN ALE maturation in a similar way to DOXO and CPT ( Fig. 4b,d ). We then tested whether HuR associates with CENPN transcripts before ALE maturation has been completed, and whether this association is decreased by DOXO and CPT. For this, we peformed RNA-immunoprecipitation using an anti-HuR antibody (3A2) followed by RT-qPCR. As expected from previous studies and validating our assay, HuR was found associated with c-fos but not gapdh transcripts ( Fig. 5e ) [37] . Importantly, HuR was associated with CENPN pre-mRNA containing the uncleaved E12 polyA site, and both DOXO and CPT treatments decreased this association ( Fig. 5e,f , ‘uncl. pA12’). The effect of CPT on HuR association with CENPN pre-mRNA containing uncleaved pA12 was about twofold stronger than the effect of DOXO, as in the case of CENPN-pA12 mRNA expression regulation ( Fig. 1h,i ). We also detected HuR association with spliced CENPN-pA12 transcripts, but this association was not decreased by DOXO and CPT ( Fig. 5e,f , ‘spliced E12’). Thus, DOXO and CPT inhibit HuR association with CENPN pre-mRNA, but not mature mRNA, in line with their effect on ALE maturation. Altogether, our data suggest that DOXO and CPT may regulate CENPN ALEs by inhibiting the association of HuR with CENPN pre-mRNA. 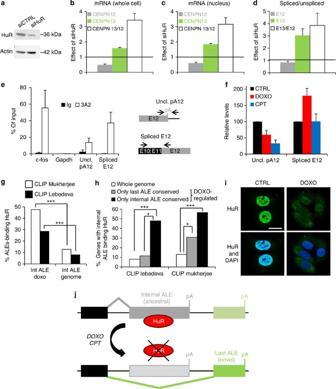Figure 5: Internal ALE repression by TOP inhibitors is mediated by HuR dissociation from pre-mRNA. (a) Western blot showing HuR depletion following siRNA transfection for 48 h. siCTRL, siRNA targeting luciferase. Representative data of three independent experiments are shown. (b–d) RT–qPCR analysis of CENPN transcripts following siRNA transfection for 48 h. Shown is the fold-effect of the siRNA targeting HuR on CENPN isoforms in whole cells (b) and nuclear fraction (c), and on the nuclear ratio of spliced to unspliced transcripts for each ALE (d). Data represent the mean±s.e.m. of three independent experiments. (e,f) RT–qPCR analysis on the indicated transcripts (see text) following RNA immunoprecipitation using an anti-HuR antibody (3A2) or control immunoglobulins (Ig). In (f), effects of drugs (6 h) on HuR association with CENPN transcripts (controls are set to 100). Data represent the mean±s.e.m. of three independent experiments. (g,h), Enrichment of HuR-binding sites in DOXO-repressed internal ALEs, compared with other internal ALEs in the genome. Two indicated data sets were analysed. *P<5.10−2and ***P<5.10−8. Test of proportions, comparing DOXO-regulated and genome-wide internal ALEs (n=62 and 2,098, respectively). (i) Effect of DOXO treatment for 6 h on HuR protein localization by immunofluorescence using the 3A2 antibody. Representative data of four independent experiments are shown. Scale bar, 5 μm. (j) Model of ALE regulation by DOXO through HuR. DOXO preferentially represses splicing of conserved internal ALEs by inducing HuR dissociation from pre-mRNA. CPT can also repress internal ALEs by the same mechanism. Exons and introns are represented by rectangles and lines, respectively. pA, polyA site. Figure 5: Internal ALE repression by TOP inhibitors is mediated by HuR dissociation from pre-mRNA. ( a ) Western blot showing HuR depletion following siRNA transfection for 48 h. siCTRL, siRNA targeting luciferase. Representative data of three independent experiments are shown. ( b–d ) RT–qPCR analysis of CENPN transcripts following siRNA transfection for 48 h. Shown is the fold-effect of the siRNA targeting HuR on CENPN isoforms in whole cells ( b ) and nuclear fraction ( c ), and on the nuclear ratio of spliced to unspliced transcripts for each ALE ( d ). Data represent the mean±s.e.m. of three independent experiments. ( e , f ) RT–qPCR analysis on the indicated transcripts (see text) following RNA immunoprecipitation using an anti-HuR antibody (3A2) or control immunoglobulins (Ig). In ( f ), effects of drugs (6 h) on HuR association with CENPN transcripts (controls are set to 100). Data represent the mean±s.e.m. of three independent experiments. ( g , h ), Enrichment of HuR-binding sites in DOXO-repressed internal ALEs, compared with other internal ALEs in the genome. Two indicated data sets were analysed. * P <5.10 −2 and *** P <5.10 −8 . Test of proportions, comparing DOXO-regulated and genome-wide internal ALEs ( n =62 and 2,098, respectively). ( i ) Effect of DOXO treatment for 6 h on HuR protein localization by immunofluorescence using the 3A2 antibody. Representative data of four independent experiments are shown. Scale bar, 5 μm. ( j ) Model of ALE regulation by DOXO through HuR. DOXO preferentially represses splicing of conserved internal ALEs by inducing HuR dissociation from pre-mRNA. CPT can also repress internal ALEs by the same mechanism. Exons and introns are represented by rectangles and lines, respectively. pA, polyA site. Full size image In the entire CENPN gene, only two HuR-binding sites were consistently found by two independent CLIP-seq studies that mapped HuR-binding sites on a genome-wide scale [37] , [38] . Remarkably, both of these sites lie in E12, and additional (potentially weaker) binding sites are also found in E12 by each CLIP-seq study ( Supplementary Fig. 6 ). To assess whether HuR may play a wider role in internal ALE repression by DOXO, we then analysed HuR-binding sites in the set of DOXO-regulated ALEs. HuR binding sites were found in ~30–50% (depending on data set) of DOXO-repressed internal ALEs, as opposed to only ~10% of non-regulated internal ALEs ( Fig. 5g ). This enrichment was still observed after normalization against exon size ( Supplementary Fig. 5b ) and was striking given that both HuR CLIP-seq analyses were done in different cell lines than our study on DOXO. The enrichment of HuR-binding sites was particularly strong for DOXO-repressed internal ALEs corresponding to ancestral last exons ( Fig. 5h , ‘only internal ALE conserved’), thus identifying HuR binding as a determinant of the preferential repression of conserved internal ALEs by DOXO ( Figs 1d and 2e ). We also validated for two other genes that HuR depletion favored the nuclear production of the last ALE like DOXO ( Supplementary Fig. 5c,d ). Finally, as expected from a previous study [43] , DOXO induced partial relocalization of HuR from the nucleus to the cytoplasm ( Fig. 5i and Supplementary Fig. 5e ). Altogether, our findings that DOXO induces dissociation of HuR from DOXO-repressed internal ALE within pre-mRNA ( Fig. 5f ), HuR depletion mimics the effect of DOXO on ALE splicing ( Fig. 5b–d ) and HuR-binding sites are enriched in DOXO-repressed internal ALEs ( Fig. 5g,h ) suggest that HuR mediates the repression of at least a subset of internal ALEs in response to DOXO ( Fig. 5j ). ALEs were identified in many human genes, but little is known about their regulation on a large scale. The regulation of ALEs depends on an interplay between pre-mRNA splicing and other nuclear processes, especially cleavage/polyadenylation and transcription termination. In this study, we show that ALEs are a major type of exons regulated by TOP inhibitors; DOXO represses a particular subset of internal ALEs corresponding to ancestrally last exons; this effect is mediated at least in part by HuR acting at the level of pre-mRNA maturation, and DOXO-regulated ALEs are involved in cell cycle regulation. These data shed new light on the regulation and function of ALEs, and identify ALEs as a novel layer of exon regulation by genotoxic agents. While internal ALEs often correspond to low-abundance, poorly conserved and truncated isoforms [9] , [10] , [11] , [12] , [13] ( Fig. 2b,e ), the set of internal ALEs repressed by DOXO is strongly enriched in a particular class identified herein as highly expressed, ancestrally last exons of genes ( Fig. 2a,b,e ). It would be interesting to identify this class of ALEs on a genome-wide scale to further determine their structural and functional properties. For example, they tend to occur in the penultimate exon of genes ( Supplementary Fig. 5f ). There may exist a selection pressure to maintain high expression of these ancestrally full-length isoforms. Their high expression may be due in part to relatively high 3′-splice site strength ( Supplementary Fig. 5g ) and/or to HuR-binding sites ( Fig. 5h ). Indeed, our findings suggest that DOXO-repressed internal ALEs depend on HuR for inclusion in mature mRNA ( Fig. 5 and Supplementary Fig. 5a–c ). Consistently, genome-wide mapping of HuR-binding sites revealed its binding to many pre-mRNAs, and HuR can regulate both splicing and polyA site use [37] , [38] , [39] , [40] , [41] , [42] . The configuration of HuR-binding sites in CENPN exon 12, with two centrally located strong binding sites and additional (potentially weaker) binding sites along the exon ( Supplementary Fig. 6 ), is consistent with the ability of HuR to cooperatively bind at multiple sites along RNA and to multimerize [44] , which could conceivably favour the recognition of this large ALE exon by various mechanisms. For example, it might bring closer the 3′-splice site and the polyA site. Alternatively, HuR binding was proposed to stabilize pre-mRNA [37] , and this would give more time for cotranscriptional splicing and polyadenylation of the internal ALE. Also interesting in this context, RNA-bound HuR can induce chromatin modifications around exons, thereby influencing cotranscriptional splicing [40] . Alternatively, HuR could locally regulate the 3′-splice site or the polyA site of exon 12, because one CLIP-seq study found HuR-binding sites in their vicinity ( Supplementary Fig. 6 ), and HuR can bind or affect the recruitment of splicing and polyadenylation factors to exons and polyA sites, respectively [39] , [41] , [42] . HuR dissociation from CENPN pre-mRNA in response to DOXO and CPT is consistent with previous evidence that HuR binding to RNA is affected by DNA damage [45] , [46] , [47] . HuR is phosphorylated by several protein kinases mediating DNA damage signalling, including Chk2, p38/MAPK, PKC and Cdk1 [46] . Furthermore, HuR dissociation from pre-mRNA in response to DOXO may reflect its partial relocalization from nucleus to cytoplasm in response to DNA damage ( Fig. 5i ) [43] , [48] , [49] . Altogether, we propose the following model ( Fig. 5j ). Internal ALEs in a subset of human pre-mRNAs depend on HuR association for inclusion in mature mRNA. In response to DNA damage, this association is inhibited, thereby decreasing the production of specific isoforms (for example, CENPN-pA12). Interestingly, in addition to CENPN that is involved in G2/M, DOXO and HuR also regulate ALEs in the KIF1B gene that regulates G2/M and apoptosis, and in the MBD1 gene involved in DNA damage checkpoint activation ( Supplementary Fig. 5c,d ) 50,51 . Meanwhile, HuR relocates to the cytoplasm, where it regulates the stability and translation of various mRNAs involved in proliferation and apoptosis through binding to 3′UTRs [36] , [47] . Thus, cell responses to DNA damage may involve the coordinated regulation of both nuclear and cytoplasmic sets of transcripts by HuR. Large-scale regulation of alternative polyadenylation and splicing are increasingly involved in cellular processes, including proliferation and genotoxic responses, respectively [1] , [2] , [3] , [4] , [5] , [6] , [7] , [8] , [16] , [19] , [20] , [21] . In this context, our data provide several advances. First, with regard to the recent finding that alternative splicing is coordinately regulated by cell cycle factors [52] , we identify a set of genes involved in M phase, more specifically the centromere–kinetochore–spindle network, which are regulated at the splicing and/or polyadenylation level by DOXO ( Table 1 ). As several splicing factors are regulated during M phase [53] , it will be interesting to determine whether these pre-mRNA maturation events are regulated during the cell cycle. Moreover, our data reveal that DOXO disrupts the CCAN complex, at least in part through the regulation of CENPN ALE isoform expression ( Fig. 3 ); this regulation adds up to the direct role of TOP-II at centromeres [54] . More generally, our data and the recent finding of CENPE splicing regulation [55] raise the possibility that the tight regulation of CCAN and kinetochore assembly during the cell cycle could be mediated in part at the level of pre-mRNA maturation. Second, while the role of ALEs and intronic polyA sites in cellular processes is only emerging [11] , [15] , with different patterns of regulation associated with proliferation depending on cell models [5] , [6] , our data establish a role of ALE regulation in cell responses to TOP inhibitors. Interestingly, the preferential repression of intragenic polyA sites by DOXO is reminiscent of the recent finding that a UV mimetic reduces the use of internal polyA sites in many yeast genes [24] . However, there are several major differences between the two observed phenomenons: most genes in yeast do not have introns; UV affects polyA sites in 35% of yeast genes, in contrast with the high specificity of DOXO effects in human cells toward evolutionarily recent last ALEs; finally, while UV inhibits cleavage/polyadenylation in both yeast [24] and human cells (through BARD1 binding to the core cleavage/polyadenylation factor CstF) [17] , [35] , CENPN ALE regulation by DOXO does not appear to be primarily mediated by BARD1 and CstF ( Supplementary Fig. 4 ). However, our data do not exclude a potential contribution of CstF or other core cleavage/polyadenylation factors to the effects of DOXO on ALEs. Another mechanism regulating intronic polyA sites is repression by the U1 snRNA, but again, DOXO effects on ALEs were much more specific than those of U1 [11] , [12] . Finally, as hnRNP H/F proteins protect p53 transcripts against polyA repression by DNA damage [18] , they might also contribute to ALE regulation. Altogether, while our data reveal a mechanism of internal ALE repression by TOP inhibitors through HuR, it is likely that DNA-damaging agents can regulate other polyA sites by other mechanisms. Third, our findings reveal both similar and different patterns of exon regulation by different genotoxic agents. The relative inability of DOXO to favour inclusion of cassette exons and internal ALEs ( Fig. 1c,d ) likely stems from its lack of inhibition of transcription elongation [23] , which mediates exon inclusion in response to CPT and UV [19] , [21] , [56] . Cassette-exon skipping and internal ALE repression are frequently induced by both DOXO and CPT [22] ( Fig. 1c,d ), suggesting a regulation by DNA damage signalling or topoisomerases themselves. In addition to splicing regulations mediated by the EWS protein and targeting several key effectors of the DNA damage response [22] , [57] , ALE regulation mediated by HuR and targeting several genes involved in DNA damage response and cell cycle (for example, CENPN , KIF1B and MBD1 ) appears as a novel pathway of regulation of pre-mRNA maturation mediating genotoxic stress responses. Other such pathways likely remain to be identified, because other splicing factors are affected by DNA-damaging agents [16] . Characterization of these pathways should help understand cell responses to different classes of genotoxic agents. Finally, this study identifies a group of evolutionarily recent last ALEs that are induced by genotoxic agents. The low expression of these novel ALEs in the absence of stress is consistent with the lower expression of nonconserved polyA sites compared with conserved ones [13] . Some of the DOXO-induced last ALEs are potential NMD targets or disrupt functional domains (for example, CENPN-pA13), suggesting that switching to the last ALE may serve to downregulate the functional ancestral isoform encoded by the internal ALE. However, CENPN-pA13 isoform depletion partially prevents CCAN disruption and G2/M block that are induced by DOXO ( Fig. 3e,f and Supplementary Fig. 3e,f ), suggesting a (potentially dominant-negative) role for this isoform in the presence of DOXO. The observation that CENPA and CENPN but not other CENP proteins are recruited to DNA breaks in response to radiations [58] raises the possibility that the CENPN-pA13 isoform might prevent kinetochore assembly at DNA breaks. More generally, it is tempting to speculate that the recent evolution of ALEs in genes involved in DNA damage response and cell cycle provides an additional layer of gene expression regulation in complex processes and organisms. Cell culture and transfection MCF-7 cells from ATCC grown in DMEM supplemented with 10% of FBS were plated at 50–75% of confluence, 48 h before drug treatments. All treatments with DOXO (2 μg ml −1 in water), CPT (1 μM in 0.1% DMSO) and vehicle (0.1% DMSO) were done for 6 h unless otherwise stated. Cells were transfected for 48 h with siRNAs (sequences in Supplementary Table 1 ) at a final concentration of 25 nM by reverse transfection using Lipofectamine RNAiMax (Invitrogen). Cells were transfected with GFP-CENPN isoform constructs in pEGFP-C1 vector using Lipofectamine LTX reagent (Invitrogen) for 24 h. The GFP-CENPN-pA12 and ΔC-ter constructs were a generous gift from A.F. Straight [30] . FACS analysis For FACS analysis, cells were fixed in 70% ethanol at 4 °C, DNA was stained for 15 min with 20 μg ml −1 propidium iodide and 1 mg ml −1 RNase A in PBS at room temperature, and FACS data were analysed using the Mod Fit software. RNA preparation and RT–(q)PCR To prepare nuclear RNA, cells were lysed for 5 min in 10 mM Tris–HCl (pH7.8); 140 mM NaCl, 1.5 mM MgCl 2 , 10 mM EDTA and 0.5% NP40 supplemented with RNase inhibitors (Invitrogen) and nuclei were pelleted at low speed. Total and nuclear RNA were extracted using TriPURE (Roche) and 1 μl of Glycoblue (Ambion) was added for RNA precipitation. Nuclear RNA was treated with DNase I (DNAfree, Ambion). Reverse transcription (RT) was performed using M-MLV (Invitrogen) and random primers. PCR was performed using GoTaq (Promega). qPCR was performed using Master SYBR Green I (Roche) on a Roche LightCycler. Primer sequences are given in Supplementary Table 2 . Full scans of gels are provided in Supplementary Fig. 7 . Western blot Total protein extracts were prepared in 50 mM Tris HCl (pH8), 400 mM NaCl, 5 mM EDTA, 1% NP40, 0.2% SDS and 1 mM DTT supplemented with protease inhibitors. Following SDS-PAGE analysis, immunoblotting was done with antibodies against HuR or Actin. Antibodies are described in Supplementary Table 3 . Full scans of blots are provided in Supplementary Fig. 8 . Immunofluorescence Cells grown on glass coverslips were fixed with 4% paraformaldehyde for 5 min, washed with PBS/20 mM glycine, permeabilized with 0.5% Triton X-100 in PBS for 5 min, washed with PBS/20 mM glycine, incubated with antibodies against CENPA, CENPH (generous gift of S.T. Liu [59] ) or HuR in PBS/3% FBS for 1 h at room temperature, washed with PBS/20 mM glycine, and incubated for 30 min at room temperature with appropriate secondary antibodies: anti-mouse IgG (H+L) Alexa Fluor 555, anti-rat IgG (H+L) Alexa Fluor 488, or anti-mouse IgG (H+L) Alexa Fluor 488 (1/1,000, Invitrogen). Cells were incubated in DNA staining solution (0.5 μg ml −1 Hoechst 33258 in PBS) for 5 min. Coverslips were washed and mounted using fluoromount medium and sealed. Image acquisition was performed using Zeiss 780 and Leica SP5 confocal microscopes. Antibodies are described in Supplementary Table 3 . Chromatin and RNA immunoprecipitation For chromatin immunoprecipitation, 1.5 million cells were crosslinked with 1% ( v / v ) formaldehyde before lysis in 50 mM Tris–HCl (pH 7.5), 150 mM KCl, 5 mM EDTA, 1% NP40, 0.1% SDS and 0.5% sodium deoxycholate supplemented with protease and phosphatase inhibitors (Roche). DNA was sonicated for 14 cycles (30 s High, 30 s wait) using a Bioruptor (Diagenode). After spinning, lysates were diluted 1/3 in lysis buffer without SDS and immunoprecipitated overnight with an antibody against Pol-II (CTD4H8, Upstate, 3 μg ml −1 ) or control mouse immunoglobulins (Santa Cruz) that were pre-incubated with Dynabeads G (Invitrogen). After five washes in immunoprecipitation buffer and two washes in 10 mM Tris–HCl (pH 7.5), 1 mM EDTA, bead/immunoprecipitate complexes were resuspended in 50 mM Tris–HCl (pH 7.5), 5 mM EDTA, 10 mM DTT, 1% SDS, reverse-crosslinked at 65 °C overnight and treated with 20 μg of proteinase K. DNA was purified using Nucleospin columns (Macherey Nagel) and analysed by qPCR. For each condition, immunoprecipitate was compared with input (aliquot of DNA before immunoprecipitation). For RNA immunoprecipitation, 3 millions cells were lysed in 25 mM Tris–HCl (pH 7.5), 150 mM KCl, 2 mM EDTA and 0.5% NP40 0.5 mM DTT supplemented with protease, phosphatase and RNase inhibitors (Invitrogen). RNA was immunoprecipitated in lysis buffer with an antibody against HuR (3A2, Santa Cruz, 6 μg ml −1 ) or control mouse immunoglobulins that were pre-incubated with Dynabeads G. After five washes in 50 mM Tris–HCl (pH7.5), 150 mM KCl, 0.5% NP40 and two washes in 10 mM Tris–HCl (pH 7.5), 1 mM EDTA, bead/immunoprecipitate complexes were resuspended in 50 mM Tris–HCl (pH 7.5), 5 mM EDTA, 10 mM DTT and 1% SDS supplemented with RNase inhibitor, and reverse-crosslinked for an hour at 70 °C. RNA was purified from immunoprecipitates and input samples using TriPURE (Roche), treated with DNase I (Ambion) and analysed by RT–qPCR. Exon-array analyses One microgram of total RNA was processed according to the manufacturer’s instructions and hybridized to GeneChip Human Exon 1.0 ST arrays (Affymetrix). The experiments, from cell treatment to array hybridization, were performed three times. Exon-array data were analysed with Expression Console (Affymetrix) to perform quality assessment and normalized using quintile normalization. Background correction and probe selection were performed as previously described, using exon annotation from the Faster DB database [22] , [60] ( http://fasterdb.lyon.unicancer.fr/ ). Global gene regulation was calculated based on exonic probes from the whole gene. The splicing index method corresponds to a comparison of gene-normalized exon intensity values between two analysed experimental conditions. We also developed a method comparing internal ALEs with the following exon. Exon-array data of each regulated exon were visualized in gene context using the exon-array visualization tool of Faster DB (Elexir), allowing to eliminate false positives and to classify exonic regulations into different types (ALE, and so on). For CPT, a top-list of 223 exons regulated by >2.2-fold ( Supplementary Data 3 ) was used for comparison with DOXO. Functional gene annotation analyses were done using the DAVID software [61] , [62] , using the human genome as a reference. Bio-informatic analysis of ALEs Two main types of internal ALEs exist: ‘skipped ALEs’ are either skipped or included as terminal exons, whereas ‘composite ALEs’ can be included as either short internal exons or long terminal exons [7] , [8] . For bio-informatic analyses ( Figs 2b–e and 5g,h ), we compared DOXO-repressed internal skipped ALEs ( n =62) with other internal skipped ALEs genome-wide (obtained from Genbank cDNAs). In Fig. 2b , only genes with at least six cDNAs ending at either ALE were analysed. In Fig. 2c , only genes with both ALEs detected in untreated cells were analysed. In Fig. 2d,e , ambiguous cases were discarded. Exon conservation ( Fig. 2e,f ) was analysed using Multiz Alignment of 46 Vertebrates [63] in the UCSC genome browser. CLIP-Seq data were analysed by mapping reads to DOXO-regulated and control internal skipped ALEs. To look for correlation between expression of DOXO-regulated ALEs and splicing/ polyadenylation factors, we used a publicly available exon-array data set on 60 human cell lines (ENCODE) [34] . In each cell line, we calculated gene-normalized expression of 89 DOXO-stimulated last ALEs and the expression level of 163 splicing/ polyadenylation factors (list available upon request). For each couple (ALE, factor), a Spearman correlation test was run; (anti-)correlation required that rho factor be more than rho min and P value be <0.05. We found 21 factors that anti-correlated (and none that correlated) with the inclusion rate of a significant number of DOXO-stimulated last ALEs (including CENPN’s). Statistical analyses For each experimental analysis, including exon-array data analyses, at least three independent experiments were performed. In figures, error bars represent the s.e.m., which is the s.d. divided by the square root of sample number. For all statistical analyses performed in this study, tests were considered significant for P ≤0.05. For exon-array analyses, a Student’s paired t -test was used. The statistical tests used in other bio-informatic analyses are indicated in figure legends. How to cite this article: Dutertre, M. et al. A recently evolved class of alternative 3′-terminal exons involved in cell cycle regulation by topoisomerase inhibitors. Nat. Commun. 5:3395 doi: 10.1038/ncomms4395 (2014). Accession codes : Exon-array data for CPT and DOXO have been deposited in the NCBI Gene Expression Omnibus under accession codes GSE21840 and GSE53474 respectively.